The DNA repair endonuclease Mus81 facilitates fast DNA replication in the absence of exogenous damage The Mus81 endonuclease resolves recombination intermediates and mediates cellular responses to exogenous replicative stress. Here, we show that Mus81 also regulates the rate of DNA replication during normal growth by promoting replication fork progression while reducing the frequency of replication initiation events. In the absence of Mus81 endonuclease activity, DNA synthesis is slowed and replication initiation events are more frequent. In addition, Mus81-deficient cells fail to recover from exposure to low doses of replication inhibitors and cell viability is dependent on the XPF endonuclease. Despite an increase in replication initiation frequency, cells lacking Mus81 use the same pool of replication origins as Mus81-expressing cells. Therefore, decelerated DNA replication in Mus81-deficient cells does not initiate from cryptic or latent origins not used during normal growth. These results indicate that Mus81 plays a key role in determining the rate of DNA replication without activating a novel group of replication origins. The accurate transmission of genetic material requires the precise regulation of DNA replication. This involves controlling the rate of DNA replication and coordinating replication initiation events throughout the genome. Cellular regulatory safeguards ensure that each position within the genome replicates precisely once during each cell cycle. To guard against perturbations of DNA replication, cells have evolved several mechanisms to preserve genomic stability. For example, cell cycle checkpoints are activated when a minimum number of perturbed replication forks are detected. If DNA synthesis within early-replicating genomic regions cannot be completed, checkpoint-signalling cascades inhibit the initiation of DNA replication in late-replicating chromosomal regions [1] . When DNA synthesis rates slow down, or replication forks encounter a lesion that prevents DNA synthesis, cells can complete the replication process by increasing the frequency of initiation events, presumably in regions adjacent to stalled replication forks [2] . The involvement of the S-phase checkpoint in initiating DNA replication emphasizes the importance of the initiation stage in ensuring genomic stability. Within eukaryotic cells, replication initiates at multiple, non-random sites called replication origins [3] , [4] . Metazoa appear to possess potential replication origins in excess (that is, more than are required for efficient replication), and, for each cell division, initiation sites are chosen anew [3] , [5] , [6] . A critical part of the choice of replication initiation sites is the binding of the mini-chromosome maintenance (MCM) helicase complex to origins to license them for replication [7] , [8] . Many licensed origins, however, do not initiate replication [9] . The apparent excess of potential origins may ensure coordination between replication, transcription and other chromatin functions [10] , [11] , [12] . The frequency of initiation can be affected by several factors including metabolic conditions (for example, nucleotide availability [13] ), developmental stage [14] and the presence of stalled replication forks. The fact that stalled replication forks can increase initiation frequency suggests that cells maintain a reservoir of unused origins that can be activated when replication is perturbed [3] , [6] . According to the terminology proposed by Mechali [6] , potential replication origins are defined as ‘flexible origins’ if they are activated at various frequencies during normal cell proliferation, or as ‘dormant origins’ (also defined as ‘cryptic origins’ or ‘latent origins’) if they are not utilized during normal growth and are only activated under distinct metabolic conditions or following cell cycle perturbations. Extra replication initiation events that occur when cell cycle progression is temporarily perturbed may arise from pre-licensed back up origins to ensure that DNA within the affected region is eventually replicated [15] , [16] , [17] , [18] , [19] , [20] . The stabilizing influence of flexible or dormant replication origins is underscored by observations in yeast that a reduced number of active origins elevates the rate of chromosome loss [21] and can trigger a cell cycle checkpoint [22] . In the absence of a cell cycle checkpoint, reduced levels of initiation can lead to gross chromosomal abnormalities [23] , [24] and DNA breakage [25] , [26] . Genomic regions with low initiation frequencies tend to be fragile [27] and DNA breaks are common in regions that replicate slowly (that is, common mammalian fragile sites [28] and replication slow zones in yeast [4] ). Although inhibition of DNA synthesis can activate the S-phase checkpoint, signalling thresholds associated with this process dictate that numerous forks must stall before the checkpoint is activated [22] . As such, mild perturbations to DNA replication decelerate replication but do not activate the checkpoint. In this way, cells are protected from the potential deleterious effects associated with checkpoint activity (that is, apoptosis and error-prone repair/recombination). We have previously shown [29] , [30] that exposures to low, non-toxic doses of replication inhibitors slow the pace of DNA synthesis and activate a specialized signalling pathway including the cancer-predisposing Bloom syndrome, RecQ helicase-like ( BLM ); Mus81 endonuclease homologue ( S. cerevisiae ) ( Mus81 ); and the ataxia telangiectasia and Rad3-related ( ATR ) kinase. Activation of this pathway initially results in DNA breaks, which are rapidly repaired by the non-homologous end-joining pathway. This reaction involves DNA-PK and X-ray repair complementing defective repair in Chinese hamster cells 4 ( XRCC4 ). Rapid repair of these DNA breaks prevents cell cycle arrest. Following the initial deceleration of DNA synthesis, replication resumes at a reduced rate without further DNA breakage. These findings suggest that transient DNA breaks induced by the inhibition of DNA replication are actively generated as damage-repair intermediates. Mus81 and BLM are involved in cellular responses to exogenously induced replicative stress. It is likely, however, that transient decelerations in DNA replication also occur under normal conditions. Here we ask whether Mus81 endonuclease plays a role in determining the rate of DNA replication during normal cellular growth. We also ask whether decreases in the rate of DNA replication are sufficient to alter replication initiation frequency and to trigger initiation from latent replication origins that are not normally utilized during unchallenged growth. In the absence of replication-perturbing agents, Mus81 promotes replication fork progression. An intact Mus81 endonuclease domain is required for a normal pace of DNA replication and for protecting cells from deleterious effects of replication inhibition (for example, a low dose of aphidicolin or depletion of XPF endonuclease). In addition, loss of Mus81 increases initiation frequency from flexible replication origins that are utilized in both Mus81-proficient and deficient cells, but does not activate novel dormant replication origins. Mus81 deficiency slows DNA synthesis To determine whether Mus81 affects replication under normal conditions (that is, in cells that are not exposed to DNA-damaging agents), we measured replication fork progression and replication initiation frequency in HCT116 cells lacking Mus81 ( Mus81 -deficient cells or Mus81 −/−) [30] , [31] . Control measurements were performed using an isogenic HCT116 cell line that carries a wild-type copy of Mus81 ( Mus81 -proficient cells or HCT116) [30] , [31] . Cell cycle profiles were similar in Mus81 -deficient and proficient cells ( Supplementary Fig. 1a,b ). We measured rates of replication fork progression by sequentially labelling cells with the thymidine analogues iodo-deoxyuridine (ldU) and chloro-deoxyuridine (CIdU). DNA fibres were then obtained from labelled cells and stretched onto microscope slides. Regions of nucleotide analogue incorporation (replication tracks) were visualized on these stretched DNA fibres using immunofluorescence, as described [30] , [32] ( Fig. 1a,b ). Using this technique, most replication tracks appeared as regions of green fluorescence (IdU incorporation) adjacent to regions of red fluorescence (CldU incorporation). This represents the fluorescent signature of replication fork progression. Lengths associated with ldU and CIdU incorporation were measured and rates of replication fork progression were calculated from these values. Fluorescent in-situ hybridization (FISH) was used to confirm these size ranges. The inclusion of a FISH signal serves an internal DNA size control. Despite the inclusion of a FISH marker, accurate comparisons of replication fork progression rates using dynamic molecular combing require that the studied samples be labelled and processed at the same experiment because minor variations in the duration of the thymidine analogue pulses can cause variations in the length of replication tracks. Comparisons among measurements obtained from separate biological replicates necessitate a common sample that can serve as a standard, as reported below. 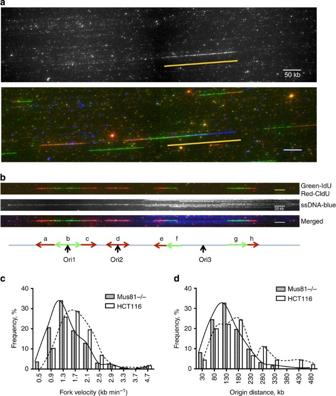Figure 1: A high frequency of replication initiation and slower replication forks inMus81-deficient cells. Cells were sequentially labelled with ldU and CIdU. Extracted DNA was then stretched on silanized microscope coverslips. Regions of DNA that contained ldU and CIdU were fluorescently labelled via immunochemistry. DNA fibres were counterstained using an antibody directed against single-stranded DNA to exclude end-fibre replication tracks from progression-rate calculations, and to ensure that origins used to calculate an inter-origin distance were on the same fibre. (a) Raw images that include a FISH signal (top, traced by a yellow line) and a merged image of FISH (blue) and replication signals (green for IdU and red for CldU). A BAC of known size was used as the FISH probe for fibre size calibration. Scale bar, 50 kb. (b) Typical replication signals (replicating DNA, top; an anti-single strand DNA (ssDNA) antibody to trace DNA fibre, middle; Merged image, blue for ssDNA, bottom). The corresponding schematic diagram is shown underneath the fluorescence images (seeSupplementary Fig. 2for more DNA fibre examples). Replication initiation events occurred during the initial IdU labelling (Ori1), during the secondary CldU labelling (Ori2) or before labelling was initiated (Ori3). Inter-origin distances were measured in fibres that contained at least two initiation events. Replication tracks that represented 20 min of DNA synthesis (a,c,e,f,g and h) were used to calculate replication fork velocity. Replication tracks that represented less than 20 min (b, d, initiated during a labelling) or that localized to the end of the DNA fibre (not showed) were not used. Scale bar, 20 kb. (c,d). Data were binned and the percentage of replication signals that corresponded to a particular range of replication-rate (c) or inter-origin distance (d) was plotted for bothMus81-proficient (HCT116) andMus81-deficient (Mus81−/−) cells.Mus81-deficient cells exhibited slower replication fork progression (c), and a higher frequency of replication initiation events (d). (c) and (d) are representative graphs from three experiments. Statistical analyses are shown inSupplementary Table 1. Figure 1: A high frequency of replication initiation and slower replication forks in Mus81 -deficient cells. Cells were sequentially labelled with ldU and CIdU. Extracted DNA was then stretched on silanized microscope coverslips. Regions of DNA that contained ldU and CIdU were fluorescently labelled via immunochemistry. DNA fibres were counterstained using an antibody directed against single-stranded DNA to exclude end-fibre replication tracks from progression-rate calculations, and to ensure that origins used to calculate an inter-origin distance were on the same fibre. ( a ) Raw images that include a FISH signal (top, traced by a yellow line) and a merged image of FISH (blue) and replication signals (green for IdU and red for CldU). A BAC of known size was used as the FISH probe for fibre size calibration. Scale bar, 50 kb. ( b ) Typical replication signals (replicating DNA, top; an anti-single strand DNA (ssDNA) antibody to trace DNA fibre, middle; Merged image, blue for ssDNA, bottom). The corresponding schematic diagram is shown underneath the fluorescence images (see Supplementary Fig. 2 for more DNA fibre examples). Replication initiation events occurred during the initial IdU labelling (Ori1), during the secondary CldU labelling (Ori2) or before labelling was initiated (Ori3). Inter-origin distances were measured in fibres that contained at least two initiation events. Replication tracks that represented 20 min of DNA synthesis (a,c,e,f,g and h) were used to calculate replication fork velocity. Replication tracks that represented less than 20 min (b, d, initiated during a labelling) or that localized to the end of the DNA fibre (not showed) were not used. Scale bar, 20 kb. ( c , d ). Data were binned and the percentage of replication signals that corresponded to a particular range of replication-rate ( c ) or inter-origin distance ( d ) was plotted for both Mus81 -proficient (HCT116) and Mus81 -deficient ( Mus81 −/−) cells. Mus81 -deficient cells exhibited slower replication fork progression ( c ), and a higher frequency of replication initiation events ( d ). ( c ) and ( d ) are representative graphs from three experiments. Statistical analyses are shown in Supplementary Table 1 . Full size image Our analyses demonstrate that during unperturbed growth, cells deficient for Mus81 replicate more slowly than Mus81 -proficient cells ( Fig. 1c and Supplementary Table 1 ). Cells lacking Mus81 had, on average, shorter replication tracks, which indicate a significantly slower DNA synthesis rate (the median rate of replication fork progression was 1.42 kb min −1 in Mus81 -deficient cells, compared with 1.74 kb min −1 in Mus81 -proficient cells ( Supplementary Table 1 ). The slower average replication fork progression in Mus81 -deficient cells could indicate either a mild but uniform overall reduction in DNA synthesis rates in all replication forks, or a substantial reduction in the pace of DNA synthesis in a group of replication forks. Mus81 deficiency increases replication initiation frequency Using this same sequential-labelling technique, distances between replication origins were also measured on stretched DNA fibres. As shown in Fig. 1b , initiation events that occurred before the first label was introduced were detected as an unlabelled region flanked by IdU-positive regions (green), which were in turn flanked by CldU-positive regions (red). Replication initiation events that occurred during the initial labelling period (IdU) were detected as an IdU-positive region flanked by CldU-positive regions. Finally, replication initiation events that occurred during the second labelling period (CldU) were detected as a CIdU-positive region flanked by unlabelled DNA. To determine whether the slow rate of DNA synthesis in Mus81 -deficient cells was accompanied by a higher frequency of initiation events, we measured inter-origin distances in both Mus81 -deficient and proficient cells. As shown in the distribution of inter-origin distances plotted in Fig. 1d , Mus81-proficient cells contained a group of fibres with longer inter-origin distances (hence the appearance of a bimodal distribution). The average inter-origin distance was significantly shorter in the Mus81 -deficient cells compared with the Mus81 -proficient controls (124.8 and 161.2 kb, respectively; Fig. 1d and Supplementary Table 1 ). These observations suggested that cells that lacked Mus81 initiated replication more frequently than isogenic cells that carried a wild-type copy of Mus81 . Fork density per Mb DNA fibre was also analysed from four random selected images for HCT116 cells and Mus81 −/− cells, respectively ( Table 1 ) and the results confirmed the inter-origin data, that is, Mus81 -deficient cells initiated DNA replication more frequently than Mus81 -proficient cells. Table 1 DNA replication fork density (forks/Mb DNA). Full size table Shorter replication tracks reflect either a slower rate of DNA synthesis or replication fork stalling, preventing DNA synthesis from proceeding during a significant length of time relative to the labelling period. To distinguish between these two possibilities, replication fork asymmetry was analysed in both Mus81 -deficient and Mus81 -proficient cells. Using the sequential-labelling technique, a stalled replication fork typically results in an asymmetric replication track (that is, tracks that emanate from a common origin but are significantly different in length) ( Fig. 2a ). A single-origin replication signal in which one side was 33% longer than the other side was defined as an asymmetric track. (For representative examples, see the rightmost fork in the fibre shown in Fig. 1b and the leftmost fork in the fibre shown in Supplementary Fig. 2c ) The frequency of asymmetric replication tracks was similar in both Mus81 -deficient and proficient cells ( Fig. 2b,c ), suggesting that Mus81 deficiency did not cause replication to stall. These observations suggest that the shorter replication tracks observed in Mus81 -deficient cells result from slower DNA synthesis rates in those cells. 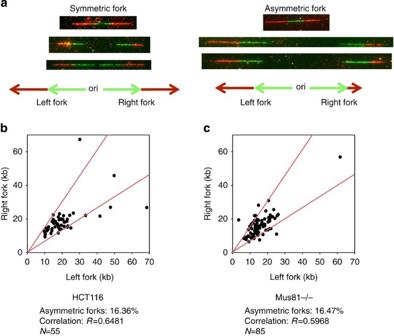Figure 2:Mus81deficiency does not trigger replication fork asymmetry. HCT116 cells were sequentially labelled with IdU (green) and CldU (red) and then subjected to single-fibre replication analyses as described in the legend toFig. 1. For each replication origin, the length of the right-fork signal was measured and plotted against the length of the left-fork signal. If the ratio between the left-fork length and the right-fork length deviated by more than 33% from 1 (that is, outside the red lines inbandc), the fork was deemed asymmetric. (a) Examples of symmetric and asymmetric forks. (b,c) The percentage of asymmetric forks was calculated for bothMus81-proficient (b) andMus81-deficient (c) cells. ForMus81-proficient andMus81-deficient cells, 55 and 85 forks were counted, respectively. Figure 2: Mus81 deficiency does not trigger replication fork asymmetry. HCT116 cells were sequentially labelled with IdU (green) and CldU (red) and then subjected to single-fibre replication analyses as described in the legend to Fig. 1 . For each replication origin, the length of the right-fork signal was measured and plotted against the length of the left-fork signal. If the ratio between the left-fork length and the right-fork length deviated by more than 33% from 1 (that is, outside the red lines in b and c ), the fork was deemed asymmetric. ( a ) Examples of symmetric and asymmetric forks. ( b , c ) The percentage of asymmetric forks was calculated for both Mus81 -proficient ( b ) and Mus81 -deficient ( c ) cells. For Mus81 -proficient and Mus81 -deficient cells, 55 and 85 forks were counted, respectively. Full size image Acute Mus81 depletion increases replication initiation rates As the cell lines used for these analyses had been propagated in culture for several months, the Mus81 phenotype (that is, the slow rate of DNA synthesis and the high rate of initiation frequency) may have resulted from long-term adaptation to the absence of Mus81 . Alternatively, these phenotypes may indicate that Mus81 is constantly involved in determining the rates of replication fork progression and replication initiation. To distinguish between these possibilities, we asked what effect an acute knockdown of Mus81 would have on DNA replication. We used siRNA to deplete Mus81 (ref. 33 ) typically achieving complete depletion 2 days following the introduction of siRNA ( Fig. 3a ). For cells exposed to siRNA directed against Mus81, we observed no significant cell cycle changes ( Supplementary Fig. 1c ). When HCT116 cells were transfected with siRNA directed against Mus81, however, DNA synthesis was significantly slower compared with cells treated with control siRNA ( Fig. 3b and Supplementary Table 2 ). This suggests that both acute and chronic depletion of Mus81 results in slower replication fork progression. In addition, cells transfected with Mus81 -specific siRNA exhibited shorter inter-origin distances, indicating an increased frequency of replication initiation events ( Fig. 3c and Supplementary Table 2 ). Similar results were obtained when the breast cancer cells MDA-MB-231 were used ( Supplementary Fig. 3 ). These results indicate that the depletion of Mus81 rapidly slows DNA synthesis and increases the frequency of replication initiation events. 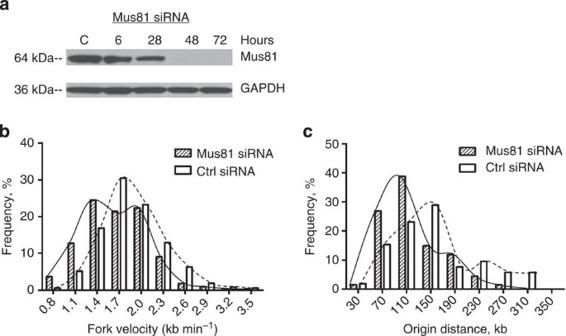Figure 3: AcuteMus81depletion triggers slower DNA synthesis and elevated initiation frequency. HCT116 cells were transfected with siRNA directed againstMus81or with control siRNA. (a) Western blot analysis showed that HCT116 cells transfected with siRNA againstMus81exhibited a marked knockdown of Mus81 protein, compared with cells transfected with control siRNA 48 and 72 h after transfection. Cells transfected with Mus81 siRNA or control siRNA for 48 h were used for single-fibre replication analyses: rates of replication fork progression (b) and inter-origin distances (c) in siRNA-treated cells. In comparisons between control- and Mus81 siRNA-treated cells, the Mann–Whitney test revealed significant differences in both replication fork velocity and inter-origin distance (Supplementary Table 2). Figure 3: Acute Mus81 depletion triggers slower DNA synthesis and elevated initiation frequency. HCT116 cells were transfected with siRNA directed against Mus81 or with control siRNA. ( a ) Western blot analysis showed that HCT116 cells transfected with siRNA against Mus81 exhibited a marked knockdown of Mus81 protein, compared with cells transfected with control siRNA 48 and 72 h after transfection. Cells transfected with Mus81 siRNA or control siRNA for 48 h were used for single-fibre replication analyses: rates of replication fork progression ( b ) and inter-origin distances ( c ) in siRNA-treated cells. In comparisons between control- and Mus81 siRNA-treated cells, the Mann–Whitney test revealed significant differences in both replication fork velocity and inter-origin distance ( Supplementary Table 2 ). Full size image Mus81 deficiency does not activate novel origins Slow replication can activate latent origins that do not initiate replication in rapidly replicating chromosomal loci [13] . We asked, therefore, whether the increase in initiation frequency that was associated with Mus81 loss-of-function also reflected the activation of latent, cryptic, unused origins. Using both Mus81 -proficient and Mus81 -deficient cell lines we mapped all replication initiation events, as described [34] . Massively parallel sequencing of newly replicated nascent DNA strands revealed strikingly similar replication-origin usage between these two cell lines ( Fig. 4 ). Similar patterns were evident in images of replication initiation patterns in individual loci (for examples, see Fig. 4a–c ), suggesting that similar genomic regions preferentially initiate DNA replication in both Mus81 -proficient and deficient cells. When the overall reads per kilobase per million aligned reads (RPKM) values were compared between the Mus81 -proficient and deficient HCT116 cells (bins that contained zero reads in both samples were excluded), Pearson correlation coefficients were 0.96 to 0.98 depending on bin size ( Fig. 4d ). Control measurements comparing two technical replicates of sequence data obtained from HCT116 cells, resulted in a Pearson correlation coefficient of 0.98. Similar trends were observed when 100-bp bins were used, although Pearson correlation coefficients were generally lower ( Fig. 4d ). Since the molecular combing data had demonstrated that Mus81 -deficient cells exhibit shorter inter-origin distances than Mus81 -proficient cells, the similar initiation patterns exhibited by the Mus81 -proficient and deficient cells imply that replication initiation events in Mus81 -deficient cells occur more frequently from the same sequences used by Mus81 -proficient cells. Therefore, the higher percentage of origins that are activated in Mus81 -deficient cells resulted from increased utilization of existing, pre-licensed flexible origins. Although the frequency of initiation was higher in Mus81 -deficient cells, we have not observed activation of genomic regions that were not utilized as replication initiation sites in Mus81 -proficient cells. 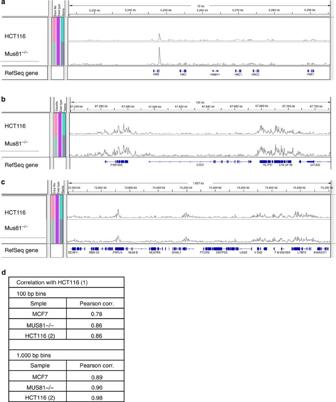Figure 4:Mus81depletion does not affect replication initiation patterns. Locations of replication initiation events were determined by massively parallel sequencing of nascent strands fromMus81-proficient HCT116 cells and from HCT116 cells that lackedMus81(designatedMus81(−/−). (a–c) Initiation profiles were visualized using the Broad Institute Integrated Genome Browser. Representative screen shots of replication initiation profiles from three genomic loci are shown at different zoom levels. These loci include (a) 72 kb from thehaemoglobin, beta (HBB)locus on Chromosome 11, (b) 195 kb from theCCCTC-binding factor(CTCF) locus on Chromosome 16, and (c) 1,857 kb from Chromosome 14. It should be noted that the genome browser images are presented on a relative scale; therefore, the sizes of the peaks (calibrated per total numbers of aligned reads in each sample) indicate that initiation events preferentially occur at particular genomic locations but do not directly correspond to absolute initiation frequencies. (d) Locations of replication initiation events were determined by massively parallel sequencing of nascent strands from: (1) HCT116 cells (two separately sequenced samples designated HCT116 (1) and HCT116 (2)), (2) HCT116 cells that lackedMus81(designatedMus81(−/−)) and (3) MCF7 cells. Locations of replication initiation sites were calculated using two bin sizes: 100 and 1,000 bp. Shown are Pearson’s correlation coefficients concerning the location of replication initiation sites for comparisons between the HCT116 (1) sample and indicated samples. Figure 4: Mus81 depletion does not affect replication initiation patterns. Locations of replication initiation events were determined by massively parallel sequencing of nascent strands from Mus81 -proficient HCT116 cells and from HCT116 cells that lacked Mus81 (designated Mus81 (−/−). ( a – c ) Initiation profiles were visualized using the Broad Institute Integrated Genome Browser. Representative screen shots of replication initiation profiles from three genomic loci are shown at different zoom levels. These loci include ( a ) 72 kb from the haemoglobin, beta (HBB) locus on Chromosome 11, ( b ) 195 kb from the CCCTC-binding factor ( CTCF ) locus on Chromosome 16, and ( c ) 1,857 kb from Chromosome 14. It should be noted that the genome browser images are presented on a relative scale; therefore, the sizes of the peaks (calibrated per total numbers of aligned reads in each sample) indicate that initiation events preferentially occur at particular genomic locations but do not directly correspond to absolute initiation frequencies. ( d ) Locations of replication initiation events were determined by massively parallel sequencing of nascent strands from: (1) HCT116 cells (two separately sequenced samples designated HCT116 (1) and HCT116 (2)), (2) HCT116 cells that lacked Mus81 (designated Mus81 (−/−)) and (3) MCF7 cells. Locations of replication initiation sites were calculated using two bin sizes: 100 and 1,000 bp. Shown are Pearson’s correlation coefficients concerning the location of replication initiation sites for comparisons between the HCT116 (1) sample and indicated samples. Full size image The endonuclease activity of Mus81 affects DNA replication Mus81 is a structure-specific endonuclease, and its endonuclease activity is required for DNA damage repair. Mus81 is part of a large protein complex that contains numerous enzymes involved in DNA repair [35] . We asked, therefore, whether it is the enzymatic activity of Mus81 that affects the rate of DNA replication. Alternatively, Mus81 could play a structural role in this process by recruiting other proteins (such as the Mus81-containing ‘super complex’) to chromatin. The endonuclease activity of Mus81 requires two aspartic-acid residues at positions 338 and 339 within the conserved nuclease domain [36] . Substituting these amino acids with alanine abolishes endonuclease activity. We used site-directed mutagenesis to reconstitute this mutation, generating an ‘endonuclease-dead’ version of Mus81 ( Fig. 5a ). We then transfected the Mus81 -deficient HCT116 cells with constructs that encoded either a wild type or endonuclease-dead version of Mus81 ( Fig. 5b ). Neither of these constructs affected cell cycle progression of Mus81 -deficient cells ( Supplementary Fig. 1d ). Complementation with the wild-type Mus81 partially restored the slow replication observed in the Mus81 -deficient cells. Expression of endonuclease-dead Mus81 resulted in slower replication fork progression and shorter inter-origin distances than expression of wild-type Mus81 ( Fig. 5c,d and Supplementary Table 3 ). This suggests that the endonuclease activity of Mus81 is involved in regulating the pace of DNA replication. 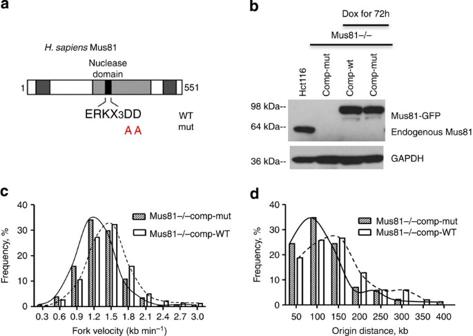Figure 5: Mus81 endonuclease activity is required to maintain replication rates. (a) Site-directed mutagenesis was used to replace two aspartic-acid residues within the conserved Mus81 nuclease domain (338 and 339) with alanine residues. (b–e) Wild type and mutant versions of Mus81 tagged with tGFP in a doxycyclin-inducible vector were introduced into HCT116Mus81−/− cells and stable cell lines were established. (b) Western blot analysis showed reproducible Mus81 expression in response to doxycycline for 72 h in these stable cell lines. (c,d) Single-fibre replication analyses were used to measure rates of replication fork progression (c) and inter-origin distances (d) in these cells after 72 h of Mus81-tGFP induction by doxycycline. Cells complemented with the wild-typeMus81exhibited slower replication fork progression compared with the rates of DNA synthesis in the parentalMus81-proficient HCT116 cells shown inFig. 1, reflecting either experimental variation or incomplete complementation byMus81. Cells expressingMus81with a mutant nuclease domain exhibited slower replication fork progression and more frequent initiation than cells expressing the wild-typeMus81. Statistical analyses are shown inSupplementary Table 3. Figure 5: Mus81 endonuclease activity is required to maintain replication rates. ( a ) Site-directed mutagenesis was used to replace two aspartic-acid residues within the conserved Mus81 nuclease domain (338 and 339) with alanine residues. ( b – e ) Wild type and mutant versions of Mus81 tagged with tGFP in a doxycyclin-inducible vector were introduced into HCT116 Mus81 −/− cells and stable cell lines were established. ( b ) Western blot analysis showed reproducible Mus81 expression in response to doxycycline for 72 h in these stable cell lines. ( c , d ) Single-fibre replication analyses were used to measure rates of replication fork progression ( c ) and inter-origin distances ( d ) in these cells after 72 h of Mus81-tGFP induction by doxycycline. Cells complemented with the wild-type Mus81 exhibited slower replication fork progression compared with the rates of DNA synthesis in the parental Mus81 -proficient HCT116 cells shown in Fig. 1 , reflecting either experimental variation or incomplete complementation by Mus81 . Cells expressing Mus81 with a mutant nuclease domain exhibited slower replication fork progression and more frequent initiation than cells expressing the wild-type Mus81 . Statistical analyses are shown in Supplementary Table 3 . Full size image Mus81 endonuclease prevents irreversible fork stalling The Mus81 endonuclease induces DNA breakage during the repair of DNA damage (for example, interstrand crosslinks and topoisomerase cleavage complexes) [33] , [37] . Mus81 converts perturbed replication forks into DNA breaks, thereby facilitating the rapid resumption of DNA replication. This avoids irreversible inhibition of DNA synthesis, DNA damage and activation of cell cycle checkpoints [30] , [38] . Mus81 also cleaves stalled replication forks that are generated by topoisomerase I (TOP1) cleavage complexes [33] and is involved in DNA breakage at common fragile sites during early mitosis [39] , [40] . We measured the frequency of DNA breaks in Mus81 -proficient and deficient cells using a comet assay. As shown in Fig. 6a , Mus81 -deficient cells exhibited similar, although somewhat lower levels of spontaneous DNA breaks than Mus81 -proficient cells. To investigate whether Mus81 endonuclease activity played a role in the recovery from perturbed replication during S-phase, we exposed cells to low doses of aphidicolin (0.5 μg ml −1 ) shown previously to slow down replication without triggering DNA damage in Mus81 -proficient cells [30] , [38] . When cells were exposed to 0.5 μg ml −1 aphidicolin for 10 min, Mus81 -proficient cells exhibited high levels of double-strand breaks ( Fig. 6b ) but the frequency of double-strand breaks did not notably change in Mus81 -deficient cells ( Fig. 6b ). 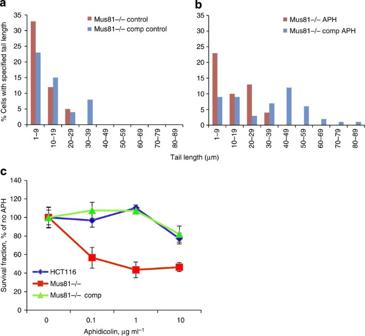Figure 6:Mus81deficiency decreases transient DNA breakage and increases sensitivity to low doses of aphidicolin. Mus81−/− (Mus81-deficient cells) andMus81-comp (Mus81−/− cells complemented with exogeneousMus81as described previously30,31) were exposed to carrier (a) or to 0.5 μg ml−1(about 1.5 μM) of aphidicolin (b) for 10 min and collected for neutral Comet assay. (c) HCT116 cells,Mus81−/− cells andMus81−/−comp cells, were treated with aphidicolin for 2 h. The survival rate of cells was determined by clonogenic assay. Figure 6: Mus81 deficiency decreases transient DNA breakage and increases sensitivity to low doses of aphidicolin. Mus81 −/− ( Mus81- deficient cells) and Mus81- comp ( Mus81 −/− cells complemented with exogeneous Mus81 as described previously [30] , [31] ) were exposed to carrier ( a ) or to 0.5 μg ml −1 (about 1.5 μM) of aphidicolin ( b ) for 10 min and collected for neutral Comet assay. ( c ) HCT116 cells, Mus81 −/− cells and Mus81 −/−comp cells, were treated with aphidicolin for 2 h. The survival rate of cells was determined by clonogenic assay. Full size image Although no significant DNA double-strand breaks were detected in Mus81 -deficient cells, colony formation assays demonstrated that Mus81 -deficient cells were markedly more sensitive to aphidicolin than Mus81 -proficient cells ( Fig. 6c ). These results suggested that the transient breaks generated by Mus81 in cells exposed to replication stress promoted cell survival by facilitating perturbed replication forks recovery. We asked, therefore, whether the endonuclease activity of Mus81 was involved in this process. Cells were labelled with IdU (green) for 10 min, then CldU (red) for 20 min. A low dose of APH was included during the CldU incubation period ( Fig. 7a ). Cells were then harvested for single DNA fibre spread analysis [29] , [30] . During APH treatment, Mus81 -proficient cells continued to replicate at a slow pace, whereas Mus81 -deficient cells fully arrested replication ( Fig. 7b ). This result is consistent with previous observations [30] . Expression of wild-type Mus81 in Mus81 -deficient cells rescued this phenotype, as a slow rate of DNA synthesis was observed during APH exposure ( Fig. 7c , left panels). When the endonuclease-dead version of Mus81 was expressed in Mus81 -deficient cells, however, replication was not restored during APH exposure, as virtually no CldU incorporation was detected ( Fig. 7c , right panels). These results demonstrate that the endonuclease activity of Mus81, in addition to regulating the pace of DNA replication, facilitates the deceleration of DNA replication and prevents irreversible inhibition of DNA replication after exposure to low doses of APH. 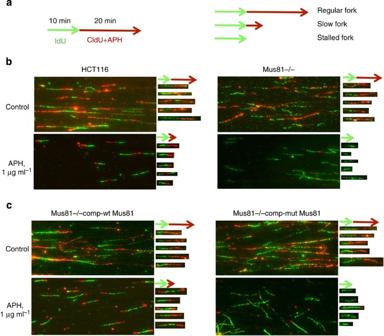Figure 7: Mus81 endonuclease activity prevents irreversible fork stalling in response to perturbed replication. (a) Cells were labelled with IdU (green) for 10 min, then CldU (red) for 20 min. A low dose of APH was included during the CldU incubation period (left). Cells were harvested for single DNA fibre spread analysis. The right schematic graph showed three typical replication tracks: regular fork, slow fork and stalled fork based on the length of red replication tracks affected by APH treatment. (b) Images of DNA fibres fromMus81-proficient (HCT116) andMus81-deficient (Mus81−/−) cells. Five representative fibres for each image were extracted and aligned to the right of their respective images. Effects of APH are shown in the bottom panels. Fibres that replicated with a similar pace during the IdU (green) and CldU (red) labelling periods exhibited a red signal that was longer than the green signal (regular fork), and most of replication forks in the control samples for both HCT116 andMus81−/− cells belong to this category (2 top panels); fibres that slowed replication during the CldU labelling period exhibited a red signal that was clearly shorter than the green signal (slow fork), and most of replication forks in APH-treated HCT116 cells belong to this category (bottom left panel); and fibres that could not recover from replication inhibition exhibited green signals and no red signals (stalled), and most of replication forks in APH-treatedMus81−/− cells belong to this category (bottom right panel). (c) Images of DNA fibres fromMus81-deficient cells that express wild-typeMus81(Mus81−/− com-wtMus81) or mutantMus81(Mus81−/−comp-muttMus81). MutantMus81lacks endonuclease activity. Effects of APH are shown in the bottom panels. Five representative fibres from APH-treated wild-typeMus81and mutantMus81samples (Fig. 7c, two bottom panels) were selected and aligned under their original images, respectively. Most of wild-typeMus81cells showed slow forks while most of mutant-typeMus81cells showed stalled forks after low dose of APH treatment. Figure 7: Mus81 endonuclease activity prevents irreversible fork stalling in response to perturbed replication. ( a ) Cells were labelled with IdU (green) for 10 min, then CldU (red) for 20 min. A low dose of APH was included during the CldU incubation period (left). Cells were harvested for single DNA fibre spread analysis. The right schematic graph showed three typical replication tracks: regular fork, slow fork and stalled fork based on the length of red replication tracks affected by APH treatment. ( b ) Images of DNA fibres from Mus81 -proficient (HCT116) and Mus81 -deficient ( Mus81 −/−) cells. Five representative fibres for each image were extracted and aligned to the right of their respective images. Effects of APH are shown in the bottom panels. Fibres that replicated with a similar pace during the IdU (green) and CldU (red) labelling periods exhibited a red signal that was longer than the green signal (regular fork), and most of replication forks in the control samples for both HCT116 and Mus81 −/− cells belong to this category (2 top panels); fibres that slowed replication during the CldU labelling period exhibited a red signal that was clearly shorter than the green signal (slow fork), and most of replication forks in APH-treated HCT116 cells belong to this category (bottom left panel); and fibres that could not recover from replication inhibition exhibited green signals and no red signals (stalled), and most of replication forks in APH-treated Mus81 −/− cells belong to this category (bottom right panel). ( c ) Images of DNA fibres from Mus81 -deficient cells that express wild-type Mus81 ( Mus81 −/− com-wt Mus81 ) or mutant Mus81 ( Mus81 −/−comp-mutt Mus81 ). Mutant Mus81 lacks endonuclease activity. Effects of APH are shown in the bottom panels. Five representative fibres from APH-treated wild-type Mus81 and mutant Mus81 samples ( Fig. 7c , two bottom panels) were selected and aligned under their original images, respectively. Most of wild-type Mus81 cells showed slow forks while most of mutant-type Mus81 cells showed stalled forks after low dose of APH treatment. Full size image The inability to recover from inhibition of DNA replication in Mus81 -deficient cells, combined with the reduced viability of Mus81 -deficient cells in response to low doses of replication inhibitors, raise the possibility that Mus81 plays a role in preventing disruptions in DNA synthesis and activation of the ATR-Chk1-mediated checkpoint. To investigate whether the ATR-Chk1 pathway was activated, we measured Chk1 phosphorylation in Mus81 -proficient and deficient cells during unchallenged growth and following exposure to APH. We observed low spontaneous levels of phosphorylation of the checkpoint kinase Chk1 on Serine 317 in Mus81 -deficient cells or in Mus81 -deficient cells complemented with endonuclease-dead Mus81 but not in Mus81 -proficient cells including Mus81 -deficient cells that were complemented with a functional Mus81. Although we observed very low levels of phosphorylation of Chk1, these phosphorylation events were reproducible and indicated that small fraction of Chk1 was persistently phosphorylated during unperturbed growth in Mus81 -deficient cells. By contrast, perturbation of DNA synthesis with aphidicolin produced a strong phosphorylation of Chk1 with enhanced Chk1 S317 phosphorylation in all cells; but the enhancement was more pronounced in Mus81 -deficient cells ( Supplementary Fig. 4 ). Intact okazaki fragment processing in Mus81 -deficient cells Recent observations in yeast suggest that the Mus81-Eme1 (essential meiotic endonuclease 1 homologue 1 ( S. pombe ) complex plays a direct role in Okazaki fragment maturation in collaboration with the FEN1 endonuclease [41] , [42] . The efficient resolution of structures generated during Okazaki fragment processing may be required for rapid DNA replication. To test this possibility, we performed a BrdU comet assay, which can detect maturation of newly replicated DNA in individual cells [43] in both Mus81 -proficient and deficient HCT116 cells. Consistent with the molecular combing data, Mus81 -deficient cells exhibited a longer tail than Mus81 -proficient cells ( Supplementary Fig. 4 ), suggesting that nascent DNA strands are on average shorter in those cells. However, the newly replicated DNA maturation rate (the rate for BrdU comet tail shortening) was similar in HCT116 cells with and without Mus81 ( Supplementary Fig. 5 ). These observations suggest that Okazaki fragment processing rates are similar in both Mus81 -proficient and deficient cells. Hence, slower Okazaki fragment maturation does not appear to be the main reason causing slower replication forks in Mus81 -deficient cells. Mus81 prevents cell death in response to XPF deficiency Our observations suggest that the endonuclease activity of Mus81 regulates both rates of DNA replication and recovery from mild DNA replication perturbations. However, Mus81 did not affect cell survival during unperturbed growth. XPF is another member of the Mus81/XPF family, which plays important roles in the repair of DNA lesions beyond nucleotide excision repair [44] . We asked, therefore, whether XPF could compensate for Mus81 deficiency during unperturbed growth. Mus81 -proficient and Mus81 -deficient HCT116 cells were transfected with siRNA directed against XPF (two times within 72 h). XPF expression was depleted 3 days after the second transfection ( Fig. 8a ). As shown in Fig. 8b , XPF depletion decreased replication fork speed in both Mus81 wild type and Mus81 -deficient HCT116 cells. Notably, however, XPF depletion by itself affected DNA replication rates to a lesser extent than Mus81 depletion, and double depletion of Mus81 and XPF did not exhibit synergistic effects. Similar changes in inter-origin distances were shown in Fig. 8c . 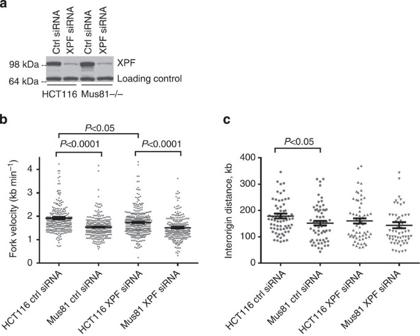Figure 8: Effects of depletion ofXPFon replication fork progression inMus81−/− cells. HCT116 andMus81−/− cells were transfected with siRNA directed againstXPFor control siRNA. (a) Western blot analysis revealed an efficient knockdown of XPF protein via siRNA treatment. (b,c) Cells were sequentially pulsed with IdU and CldU for 20 min, respectively, before harvesting for DNA combing. Scatter plot was used to show the distribution of replication fork speed (b) and inter-origin distance (c). Median with interquartile range was shown for the scatter plot. Mann–Whitney test was used for the statistical analysis. A few extreme numbers (>4.5 kb min−1for fork speed, >400 kb for origin distance) were not shown for a better resolution of the scatter plot. Statistical analyses were shown inSupplementary Table 4. Figure 8: Effects of depletion of XPF on replication fork progression in Mus81 −/− cells. HCT116 and Mus81 −/− cells were transfected with siRNA directed against XPF or control siRNA. ( a ) Western blot analysis revealed an efficient knockdown of XPF protein via siRNA treatment. ( b , c ) Cells were sequentially pulsed with IdU and CldU for 20 min, respectively, before harvesting for DNA combing. Scatter plot was used to show the distribution of replication fork speed ( b ) and inter-origin distance ( c ). Median with interquartile range was shown for the scatter plot. Mann–Whitney test was used for the statistical analysis. A few extreme numbers (>4.5 kb min −1 for fork speed, >400 kb for origin distance) were not shown for a better resolution of the scatter plot. Statistical analyses were shown in Supplementary Table 4 . Full size image By contrast, when Mus81 -deficient cells were treated with XPF siRNA, they exhibited a marked increase in sub G1 or apoptotic cells as measured by flow cytometry analyses ( Fig. 9a,b and Supplementary Table 5 ). Annexin V and TUNEL apoptotic assay confirmed that there were more apoptotic cells in Mus81 -deficient cells when XPF was depleted ( Fig. 9c , Supplementary Fig. 6 ). In agreement, clonogenic assays showed that depletion of XPF markedly decreased the survival of HCT116 cells. This effect was more pronounced in Mus81 -deficient cells ( Fig. 9d ). These results suggest that XPF may act in concert with Mus81 to prevent the formation of deleterious DNA lesions. These results also demonstrate that at least one of the two endonucleases is required for the normal progression of DNA synthesis during an unperturbed cell cycle, and that XPF may promote cell survival in the absence of Mus81 during unperturbed growth. 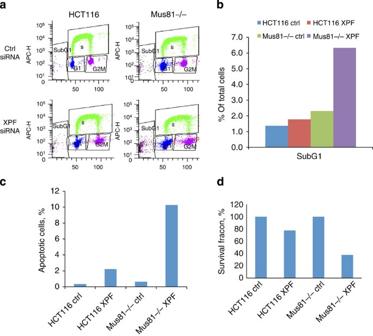Figure 9: Effects of depletion ofXPFonMus81−/− cell survival. HCT116 andMus81−/− cells were transfected with control siRNA orXPFsiRNA as described inFig. 8. (a) Cell cycle analysis by FACS. Cells were pulse-labelled with EdU for 45 min before harvesting. Cell cycle was tested with a Click-iT EdU kit by FACS. Examples of bivariate FACS were shown and percentage of cells in each cell cycle was shown inSupplementary Table 5. (b) Histogram of percentage of subG1 from (a). (c) The % of apoptotic cells was measured by TUNEL assay. Cells were transfected with control siRNA orXPFsiRNA twice with 72 h interval and collected 72 h after the second transfection. TUNEL-positive cells were analysed by FACS (seeSupplementary Fig. 6Bfor the FACS dot plots). (d) Clonogenic assays. Twenty-four hours after the second siRNA transfection, cells were seeded into six-well plates at 50, 250 or 1,000 cells per well. Two weeks later, cells were fixed and stained to count the colonies. Figure 9: Effects of depletion of XPF on Mus81 −/− cell survival. HCT116 and Mus81 −/− cells were transfected with control siRNA or XPF siRNA as described in Fig. 8 . ( a ) Cell cycle analysis by FACS. Cells were pulse-labelled with EdU for 45 min before harvesting. Cell cycle was tested with a Click-iT EdU kit by FACS. Examples of bivariate FACS were shown and percentage of cells in each cell cycle was shown in Supplementary Table 5 . ( b ) Histogram of percentage of subG1 from ( a ). ( c ) The % of apoptotic cells was measured by TUNEL assay. Cells were transfected with control siRNA or XPF siRNA twice with 72 h interval and collected 72 h after the second transfection. TUNEL-positive cells were analysed by FACS (see Supplementary Fig. 6B for the FACS dot plots). ( d ) Clonogenic assays. Twenty-four hours after the second siRNA transfection, cells were seeded into six-well plates at 50, 250 or 1,000 cells per well. Two weeks later, cells were fixed and stained to count the colonies. Full size image Mus81 plays an important role in preserving genomic integrity by promoting homologous recombination-mediated repair, mitotic recombination and the resolution of DNA lesions including interstrand crosslinks [31] , [37] , [45] , [46] , [47] . Importantly, Mus81 plays an active role in generating DNA breaks in cells exposed to campthotecin [33] and in the cellular response to replication inhibitors, facilitating breaks at common fragile sites during early mitosis [39] , [40] . When cells encounter conditions that slow DNA replication such as exposure to DNA polymerase inhibitors, Mus81 in coordination with BLM and ATR converts stalled replication forks into double-stranded DNA breaks. These breaks are subsequently repaired via non-homologous end joining to prevent the activation of DNA-damage checkpoints and allow cells to resume replication [29] . While all the above studies suggest a role for Mus81 endonuclease in the resolution of lesions resulting from perturbation of DNA replication, here we show that unchallenged Mus81 -deficient cancer cells exhibited slower rates of DNA replication and higher frequencies of replication initiation events. This suggests that Mus81 also plays a role during unperturbed S-phase to regulate DNA replication in the absence of DNA-damaging agents and stimuli that slow replication. Mus81 -deficient cells exhibit a higher frequency of initiation events and slow DNA replication. While these two phenomena are linked, the causal relationship between them is unclear: Loss of Mus81 activity may either result in slow replication, increasing initiation frequency as a secondary consequence, or loss of Mus81 can facilitate initiation, slowing replication indirectly. Our observations are consistent with both possibilities. Notably, the distribution of replication fork progression rates in Mus81 -deficient cells could indicate either an overall mild but uniform reduction in the pace of DNA synthesis or a marked reduction in DNA synthesis rates that is limited to a subset of replication forks. If only a subset of replication forks is markedly affected, these data are consistent with a role for Mus81 in resolving lesions that occur in a small but significant fraction of replication forks during S-phase such as replication fork reversal (as shown in the working model illustrated in Supplementary Fig. 7 ). This hypothesis is consistent with the known substrate specificity of Mus81 endonuclease activity, since stalled replication forks ( Supplementary Fig. 7b ) and/or reversed forks ( Supplementary Fig. 7g ) can serve as potential substrates. Interestingly, our studies suggest that the endonuclease activity of Mus81 is required for setting the pace of DNA replication during unperturbed growth as well as for the response to replication inhibitors, eliminating the possibility that Mus81 primarily provides a scaffold to recruit other proteins that regulate replication fork progression. What role can an endonuclease play in setting the pace of DNA replication? In yeast, the Mus81-Eme1 (essential meiotic endonuclease 1 homologue 1 ( S. pombe ) complex plays a direct role in Okazaki fragment maturation in collaboration with the FEN1 endonuclease [41] , [42] . In mammals, Mus81 binds late-replicating loci during early mitosis and participates in the expression of fragility at common fragile sites [39] , [40] . We found that Okazaki fragment processing efficiency was similar in Mus81 -deficient and proficient human cells, suggesting that the slower DNA replication forks in Mus81 -deficient cells could not be primarily attributed to changes in Okazaki fragment processing. As the endonuclease activity of Mus81 is required to maintain the normal rate of replication fork progression, our data suggest that Mus81-mediated DNA cleavage is required to resolve a lesion that occurs at a small but significant fraction of replication forks. Combined with the reported increase in replication fork reversal frequency in the absence of exogenous stress in Mus81 -deficient cells [48] , our data are in line with a role for Mus81 in resolving low-frequency reversed forks during unperturbed growth (see Supplementary Fig. 7 for a working model describing this hypothesis). Such a role might be critical for countering the deleterious effects of increased DNA replication fork reversal when DNA replication decelerates. An increased frequency of reversed replication forks ( Supplementary Fig. 7f ) might underlie the slow rate of DNA replication in Mus81 −/− cells under normal cell growth condition. A role for replication checkpoint proteins in regulating the pace of DNA replication was observed for ATR kinase, which suppresses overactivation of replication origins [49] , [50] via the checkpoint kinase 1 (CHEK1—Chk1) [51] , [52] . It is possible that the very limited phosphorylation of Chk1 on Serine 317 is involved in the slow replication phenotype observed in Mus81 -deficient cells during unperturbed growth. However, cell cycle checkpoints mediated by Chk1 phosphorylation following perturbation of DNA synthesis can inhibit initiation of DNA replication [51] , [52] , a phenomenon that was not observed in our study. In addition, the extent of phosphorylation observed during unperturbed replication was significantly lower than the phosphorylation typically exhibited in cells treated with APH, suggesting that the known S-phase checkpoint that involves massive Chk1 phosphorylation on Serine 317 and inhibition of initiation of DNA replication could not provide a sole explanation for the observed slow replication, frequent initiation phenotype of Mus81 -depleted cells. Other complementary or parallel pathways might involve slowing replication while activating compensatory initiation. It is also important to note that since our study was performed in cancer cells (HCT116 and MDA-MB-213) we cannot rule out the possibility that the low levels of Ser317 phosphorylation and the observed response to Mus81 deficiency reflect the transformed nature of those cells. The two structure-specific endonucleases, Mus81 and XPF, form dynamic heterodimers that exhibit partially overlapping but distinct substrate specificity [53] , [54] . Recent studies have revealed a partial overlap in homologous recombination-mediated repair functions of Mus81 and XPF following induction of double-stranded DNA breakage [55] . We report here that Mus81 protected cells from cell death in the absence of the XPF endonuclease, suggesting that Mus81 could function as a backup for XPF activity (and vice versa) during unperturbed growth. The overlapping functions of the two endonucleases can underlie the relatively mild phenotype observed for Mus81 depletion. A complementary role of XPF could also account for the variability observed in the phenotype of Mus81 depletion in other cells. For example, Mus81 -depleted Jeff, MRC5-SV and HeLa cells show no replication fork stalling and no changes in replication fork speed, Mus81 -depleted U2OS cells exhibit replication fork stalling [39] , [40] , [56] . Conversely, cells require Mus81 to recover from replication inhibition following exposure to low doses of polymerase inhibitors [30] and topoisomerase inhibitors [33] . DNA lesions that form after mild perturbation of DNA replication may be impervious to XPF-mediated repair because they are too numerous, or because they are structurally incompatible. One speculative possibility is that replication lesions formed during unperturbed growth contain structures that can be recognized by both Mus81 and XPF (for example, ‘splayed arms’ that include an extended single-stranded DNA portion [53] ), whereas structures formed following inhibition of DNA polymerases or DNA topoisomerases can predominantly be recognized by Mus81 (for example, replication forks with very short ssDNA regions [53] ). Another possibility is that replication lesions that form during unperturbed growth could be repaired by single-strand annealing, which can be catalysed by either Mus81 or XPF. In contrast, replication lesions that form after exposure to low doses of replication inhibitors require the resolution of replication forks or D-loops (via synthesis-dependent strand annealing), which can only be catalysed by Mus81 (ref. 53 ). During each cell cycle only a subset of replication origins is used to replicate the eukaryotic genome [57] . Origins are selected anew each cycle [5] and slow replication can lead to the activation of a larger subset of origins, called ‘dormant origins’ [38] , [58] , [59] , [60] . Single-fibre analyses per se cannot resolve whether activated dormant origins are selected from the pool of origins that are also activated during unperturbed growth, or if cells contain a class of latent, cryptic replication origins that are not used during normal growth but are only activated to rescue DNA replication when fork progression is perturbed (for example, during replication stress) [6] . For example, at the Chinese hamster AMPD2 locus, origins that do not initiate replication during normal growth are activated when the concentration of nucleotide precursors is reduced [13] . The nascent strand sequencing results described here revealed that the same pool of DNA sequences initiated DNA replication in the slower-replicating Mus81 -deficient cells and in the faster-replicating Mus81 -proficient cells. These data support the notion that slow replication is accompanied by higher frequencies of flexible-origin activation (that is, a greater utilization of pre-licensed origins). It is likely that the flexible origins activated at a higher frequency in Mus81 -deficient cells represent origins that are normally activated later in the S-phase of the cell cycle in Mus81 -proficient cells. This point could be investigated directly once data on replication timing in HCT116 cells become available. Our data show that Mus81 depletion does not lead to the use of novel DNA sequences, which do not initiate replication in Mus81 -depleted cells, as replication origins. However, our observations do not preclude the possibility that such latent, cryptic origins exist, and that such origins can be activated under more extreme circumstances (for example, DNA damage or chromatin reprogramming during differentiation). Cells and culture conditions HCT116 and HCT116 Mus81 −/− cells [31] were grown in Dulbecco Modified Eagle’s medium (Invitrogen), whereas MDA-MB-231 cells were grown in RPMI 1640 medium. Both media were supplemented with 10% heat-inactivated fetal calf serum. APH doses were calibrated based on a survival curve [30] to correspond to a 40% survival. DNA replication profiling by molecular combing Asynchronous exponentially growing cells were labelled with 20 μmol l −1 IdU for 20 min. They were then washed in phosphate-buffered saline (PBS) and subsequently labelled with 50 μmol l −1 CldU for 20 min, then cells were chased with of 200 μmol l −1 of thymidine for 60–90 min. Cells were trypsinized and resuspended in PBS. Cells were then embedded in pulsed-field gel electrophoresis agarose plugs to prepare high-molecular-weight genomic DNA. After proteinase K digestion, agarose plugs were washed with TE buffer. Agarose plugs were then melted in 100 mmol l −1 MES (pH 6.5) and digested using 2 μl of β-agarose (Biolabs). The DNA solution was poured into a Teflon reservoir and DNA was combed onto silanized coverslips (Microsurfaces) using a combing machine. Samples have included a BAC as a molecular marker, allowing us to convert labelled signal length (in microns) to fibre length (in kb) as molecular combing was previously shown to uniform stretching [32] , [60] , [61] . Uniform stretching was confirmed by the uniform length of the stretched marker DNA. Coverslips were visually examined for DNA density and fibre length by a preliminary staining with YoYo1 (invitrogen). Sample preparations containing fibres that were mostly shorter than 200 kb or DNA concentration was too low or too high were discarded. The average fibre length in our studies is about 400 kb. For slide preparations that contained long fibres with appropriate density, coverslips with combed DNA were incubated at 60 °C for 2 h and denatured in 0.5 N NaOH for 20 min. IdU was detected using a mouse antibody directed against BrdU (IgG1, Becton Dickinson, cat.347580, 1:25). CldU was detected using a rat antibody directed against BrdU (Accurate chemical, cat. OBT0030, 1:50). Single-strand DNA (ssDNA) was detected using a mouse antibody directed against ssDNA (IgG 2a, Chemicon, cat. MAB3034, 1:100). Coverslips with DNA were incubated with primary antibodies for 1 h at room temperature. After washes, samples were incubated with secondary antibodies for 45 min. Secondary antibodies included Alexa Fluor 594 donkey antibody directed against rat (A21209, 1:100), Alexa Fluor 488 goat antibody directed against mouse IgG1 (γ1) (A-21121, Invitrogen, 1:100) and Alexa Fluor 647 goat antibody directed against mouse IgG2a (γ2a) (A21241, Invitrogen, 1:100). Slides were scanned with a BD pathway 855 controlled by AttoVision (Becton Dickinson). Fluorescent signals were measured using ImageJ (from the National Cancer Institute) with custom-made modifications. Only replication signals from high-quality ssDNA (not from DNA bundles, not located at the end of a strand) were selected for analyses. Signals were marked for evaluation by ‘blind’ measurers (not knowing which samples they were measuring); signal length was measured using the Image J software followed by automatic compilation of signal lengths into an Excel worksheet. Fork velocities and origin distances were calculated using Excel with a constant of 2 kb μm −1 . Replication fork velocities were calculated using elongating fork signals only (initiating forks were eliminated; see a recent review [62] for a discussion of good practices in dynamic molecular combing). Experiments were performed at least in duplicate using independent biological isolations of DNA fibres for each experimental condition. Statistical analysis was performed in Prism 5 or 6 (GraphPad software) using the non-parametric Mann–Whitney rank sum test. Normality of distributions was assessed using the Kolmogorov–Smirnov test. Neutral comet assay Neutral comet assay was performed using the CometAssay Kit (Trevigen) following the manufacturer’s protocol. In brief, cells were collected and suspended in low-melting-point agarose and applied to CometSlides. Then cells were lysed in lysis solution and were electrophoresed in TBE. The samples were then fixed in 70% (v/v) ethanol and dried overnight before staining with SyBr Green (Molecular Probes, Eugene, OR) to visualize cellular DNA. Images of nuclei were captured using a CCD camera (Roter Scientific; Cool SNAP FX) with epifluorescence microscopy (Olympus; IX70) using a × 20 objective lens. For each sample, 50 cells were scored for tail length. Tail length was manually measured using IPLab software. Mus81 siRNA and XPF siRNA transfection and western blotting HCT116 cells were transfected with non-targeting control siRNA (Dharmacon, D-001810-1), Mus81 siRNA (Dharmacon, L-016143-01) or XPF siRNA (Dharmacon, L-019946-00) with DharmaFECT 2 siRNA Transfection Reagent (Dharmacon, T-2002) according to the manufacturer’s protocol. All siRNA transfection other than noted in the figure legends were done twice with a 72 h interval, and cells were harvested for 3 days after the second transfection. Whole-cell lysates by 1 × SDS loading buffer were used for western blot with an anti-Mus81 antibody (Abcam, ab14387, 1:2,000) and anti-XPF antibody (Lab vision Ab1, clone 219, 1:500) to verify the knockdown efficiency of Mus81 siRNA and XPF siRNA. Phospho-Chk1 (Ser317) and total Chk1 antibodies were purchased from Cell Signalling (#2344, 1:1,000 and #2345, 1:1,000). GAPDH (Gene Tex, GTX627408, 1:5,000) and PCNA (Santa Cruz Biotech, sc-7907, 1:2,000) antibodies were used as loading controls. Cell cycle analysis Cells were pulse labelled with 10 μM EdU for 45 min before harvest. EdU staining using the Click-iT EdU kit (Invitrogen, C10424) was performed according to the manufacturer’s protocol. DAPI was used for DNA staining. For cells without thymidine analogue incorporation, PI was used for DNA staining. BD LSRFortessa cell analyzer with FACSDiva software was used for cell cycle analysis. Plasmid constructs and site-directed mutagenesis Mus81 cDNA was purchased from Origene (RG203373). QuikChange II kit (Stratagene, 200523) was used to introduce the mutations into Mus81 (D338A and D339A) as described [63] with the following primers: sense primer was 5′-gcgcaagcgactggctgccctttgcagcagca-3′, and the reverse primer was 5′-tgctgctgcaaagggcagccagtcgcttgcgc-3′. Then wild type and mutant Mus81tGFP cDNA were subcloned into Tet-On 3G Inducible Expression System (Clontech, 631168) and transfected into Mus81 -deficient HCT116 to establish stable cell lines. Clonogenic assay After XPF siRNA treatment, cells were plated at a density of 50, 250 and 1,000 per well in six-well plates and incubated for 12 days to allow formation of colonies. Cells were fixed with methanol, stained with 0.1% Commassie blue for 30 min and washed with distilled water. Colonies were counted after air-drying. Plating efficiency (PE) was defined as the number of colonies counted/the number of cells seeded. The survival fraction (SF) was calculated as: PE treated /PE untreated × 100. Nascent strand abundance assay Genomic and nascent strand DNA samples were isolated from Mus81 -proficient and Mus81 -deficient cells as described [34] , [64] , [65] with some modifications. Nascent DNA samples were loaded onto a neutral 5–30% sucrose gradient in TNE. Gradients were centrifuged at 21,000 r.p.m. for 20 h. Fractions that contained DNA fragments of 400–600 bp were pooled, dialysed against TE and precipitated. The sample was resuspended in DEPC water and was digested overnight at 37 °C with lambda exonuclease. Samples were heated to 95 °C for 10 min, ethanol precipitated and resuspended in 50 μl of sterile water. Nascent strands were random-primed using the Klenow and DNA Prime Labelling System (Invitrogen). Double-stranded nascent DNA (1 μg) was sequenced using the Illumnia genome analyzer II (Solexa). Sheared genomic DNA was sequenced as a control. Integrative genomics viewer tracks are reads per kilobase per million aligned reads (RPKM) values for nascent strand reads binned in 100 bp. Values were smoothed using a Gaussian smoothing algorithm with a window size of seven bins. RPKM values were normalized for copy-number variation using regional copy-variation values that were derived from our previous study of HCT116 cells using the Agilent aCGH 4 × 44 microarray ( http://discover.nci.nih.gov ). Pearson’s correlation coefficients between the binned and smoothed RPKM values across the entire genome were computed for HCT116 versus MUS81 -deficient cells. To avoid correlation skew, bins that were empty in both samples were excluded from the correlation calculation. BrdU comet assay The BrdU comet assay was performed as previously described [43] . In brief, HCT116 and Mus81 −/− HCT116 cells were pulsed with 100 μM of BrdU for 30 min, then harvested immediately (0 h) or chased for 1 or 6 h in pre-warmed fresh medium without BrdU. Cells were collected and the cell pellet was resuspended in cold PBS. An alkaline assay was performed according to the manufacturer’s instruction (Trevigen, 4250-050-K). Following electrophoresis, the gels were neutralized by 0.4 M Tris HCl and washed with PBS before immunostaining. The BrdU-labelled nascent DNA was detected by a mouse anti-BrdU antibody (Becton Dickinson, cat.347580, 1:10), then goat anti-mouse IgG conjugated with Alexa 488 (Invitrogen, A-21121, 1:100). The gels were then counterstained with DAPI. The samples were then dried according to the manufacturer’s instruction (Trevigen, 4250-050-K). Images were taken by a BD pathway 855 microscope controlled by AttoVision (Becton Dickinson) with × 10 or × 20 objective lens. Images were analysed by CometScore software (TriTeK). Apoptosis: Annexin V assay and TUNEL assay Annexin V kit was from Becton Dickinson (#556547) and the assays were performed as described in the manufacturer’s instructions with minor modifications. Cells were kept on ice following trypsin-mediated detachment to avoid cell death. TUNEL assay was performed as described in the manufacturer’s instructions (#11684795910, Roche). Accession codes of NGS : GSE28911 . How to cite this article: Fu, H. et al. The DNA repair endonuclease Mus81 facilitates fast DNA replication in the absence of exogenous damage. Nat. Commun. 6:6746 doi: 10.1038/ncomms7746 (2015).